Direct synthesis of formic acid from carbon dioxide by hydrogenation in acidic media The chemical transformation of carbon dioxide into useful products becomes increasingly important as CO 2 levels in the atmosphere continue to rise as a consequence of human activities. In this article we describe the direct hydrogenation of CO 2 into formic acid using a homogeneous ruthenium catalyst, in aqueous solution and in dimethyl sulphoxide (DMSO), without any additives. In water, at 40 °C, 0.2 M formic acid can be obtained under 200 bar, however, in DMSO the same catalyst affords 1.9 M formic acid. In both solvents the catalysts can be reused multiple times without a decrease in activity. Worldwide demand for formic acid continues to grow, especially in the context of a renewable energy hydrogen carrier, and its production from CO 2 without base, via the direct catalytic carbon dioxide hydrogenation, is considerably more sustainable than the existing routes. Concerns over carbon dioxide levels in the atmosphere, which have reached ca . 400 p.p.m. [1] , [2] , are leading to political targets and scientific/technological efforts to reduce CO 2 emissions and to capture CO 2 and store it within porous rock formations [3] , [4] , [5] , [6] . Converting CO 2 into useful feedstock chemicals and fuels represents another important strategy that not only removes CO 2 from the atmosphere, but also reduces dependence on petrochemicals [7] , [8] . In this context much progress has been made in recent years and several reactions have been commercialized. Examples of products now derived from CO 2 include urea, salicylic acid and polyols [3] . Recently, a company in Iceland started using renewable energy to convert CO 2 into methanol, in the region of 1,600 T per year [9] . However, human activity contributes ~35 GT of CO 2 to the atmosphere per year and there is clearly a considerable gap between the amount of CO 2 produced and the amount consumed. Ideally a multitude of chemical products should be derived from CO 2 (ref. 10 ) and an important one, as it may be employed as both a feedstock chemical and a fuel, is formic acid. Currently worldwide production of formic acid, obtained from the combination of methanol and carbon monoxide with a strong base, is in the order of 800,000 T per year and is used in the textile industry, cleaning and as a preservative, to name a few. Demand could increase considerably due to the development of efficient formic acid dehydrogenation catalysts that could find widespread application within the context of a hydrogen economy [11] . Today, with the exception of fossil fuels, practical hydrogen storage systems use pressurized bottles or cryogenic conditions [12] . As formic acid (HCOOH) has a volumetric hydrogen density of 53 g of H 2 per liter, a low-toxicity and is a liquid under ambient conditions, it is an ideal hydrogen storage material for certain applications [13] , [14] . Hydrogen production from formic acid has been achieved with a variety of homogeneous and heterogeneous catalysts [15] , [16] . Although most catalysts are based on noble metals, recent complexes based on iron (a cheap and abundant element) highlight the validity of such systems within the context of a hydrogen economy [17] . The concept of the hydrogen storage in the form of formic acid would, however, be even more attractive should a viable catalyst for the reverse reaction become available, that is, a catalyst that reduces carbon dioxide with hydrogen and in the absence of a base [18] , [19] , [20] , [21] , [22] ( Fig. 1 ). 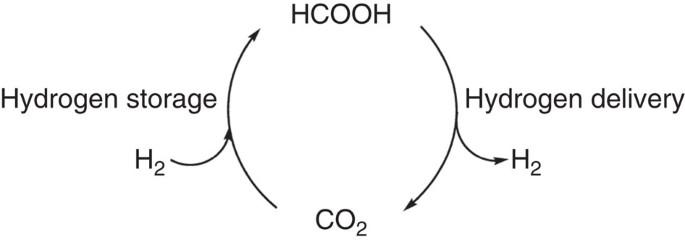Figure 1: The formic acid/carbon dioxide cycle for hydrogen storage.  Figure 1: The formic acid/carbon dioxide cycle for hydrogen storage. Full size image Several catalysts are available for both reactions, and in general, hydrogen production or consumption is controlled by the pH of the solution [23] , [24] , [25] , [26] . However, the conversion of carbon dioxide into formic acid is difficult owing to the high kinetic and thermodynamic stability of CO 2 . The gas phase reaction has a positive ΔG value because of an entropic contribution (ΔG 0 =+33 KJ mol −1 ), and the formation of formic acid is more favourable in aqueous solution (ΔG 0 =−4 KJ mol −1 ) (ref. 20 ). For reactions performed in water, the CO 2 /H 2 CO 3 /HCO 3 − equilibrium, as well as the second deprotonation to CO 3 2− , must be taken into account ( Supplementary Fig. 1 ). From these equilibria and the kinetic studies performed on the hydrogenation of bicarbonates at different pH values [27] it is apparent that the reaction is favourable in basic media, conditions where the actual substrate is HCO 3 − (ΔG 0 =−35 KJ mol −1 ) or CO 3 2− . In contrast to the direct reaction of H 2 with CO 2 , the hydrogenation of carbonate and bicarbonate are well-established reactions [28] , [29] , [30] that have been achieved in a wide variety of organic solvents, ionic liquids, water and supercritical CO 2 (ref. 20 ). Currently, catalysts that show high activity in the hydrogenation of CO 2 require additives such as bases [31] , [32] , including amines [33] or buffers [34] , [35] , producing formate salts. Ogo et al . [34] , [35] were able to produce formic acid (0.06 M) from the direct reaction of H 2 with CO 2 in an acidic buffer. The presence of base also complicates the separation of formic acid from the reaction mixture although ingenious approaches have been developed to overcome these complications [30] , [36] . Herein, we describe a homogeneous ruthenium catalyst that hydrogenates CO 2 to formic acid in acidic media, without the need of any bases, amines or buffers. In aqueous solution, 0.2 M formic acid can be obtained, in dimethyl sulphoxide (DMSO) the ruthenium(II) phosphine catalyst provides 1.9 M formic acid. Direct carbon dioxide hydrogenation in water In our initial studies the hydrogenation of CO 2 was explored in acidic aqueous solutions using ruthenium(II) or rhodium(I) catalysts with water soluble phosphine ligands, that is, 1,3,5-triaza-7-phosphaadamantane (PTA), 3-methyl-1,3,5- triaza-7-phosphaadamantane (MePTA), meta-monosulphonated triphenylphosphine (TPPMS) and meta-trisulphonated triphenylphosphine (TPPTS; Supplementary Table 1 ). From these studies [RuCl 2 (PTA) 4 ] was found to be the most active catalyst affording formic acid as the only product under the reaction conditions (at the end of the reaction the pH of the solution is 2.70, Fig. 2 and Supplementary Fig. 2 ). The ruthenium catalysts were typically 10 times more active than the rhodium analogues and the highest yields were obtained for complexes containing PTA-type ligands, that is, similar activities were observed for the PTA and MePTA ligands, whereas complexes with TPPMS and TPPTS were less active. 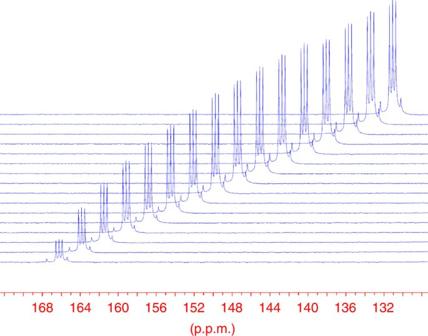Figure 2:13C NMR signals of DCOOD in the hydrogenation reactions of CO2into formic acid in D2O. [RuCl2(PTA)4] (2.76 mM) was dissolved in D2O (2 ml) under N2atmosphere in a medium pressure sapphire NMR tube. This solution was pressurized at room temperature to 50 bar with CO2and completed to 100 bar with H2. The system was heated to 60 °C and the reaction was followed by13C NMR (100 MHz) spectroscopy. The figure shows the evolution of the13C NMR signals of DCOOD at 166.3 p.p.m. (time difference between spectra Δt=189 min). The triplet signal of the formic acid is due to the exchange of the hydrogen to deuterium in HCOOH (as D2O was used as solvent). Reaction time: 148 h. The reaction conditions were optimized for [RuCl 2 (PTA) 4 ] to improve performance and the dependence of the catalyst concentration, pressure, P (H 2 )/ P (CO 2 ) ratio ( Table 1 ) and temperature ( Supplementary Table 2 ) on formic acid production was elucidated. Figure 2: 13 C NMR signals of D C OOD in the hydrogenation reactions of CO 2 into formic acid in D 2 O. [RuCl 2 (PTA) 4 ] (2.76 mM) was dissolved in D 2 O (2 ml) under N 2 atmosphere in a medium pressure sapphire NMR tube. This solution was pressurized at room temperature to 50 bar with CO 2 and completed to 100 bar with H 2 . The system was heated to 60 °C and the reaction was followed by 13 C NMR (100 MHz) spectroscopy. The figure shows the evolution of the 13 C NMR signals of D C OOD at 166.3 p.p.m. (time difference between spectra Δ t =189 min). The triplet signal of the formic acid is due to the exchange of the hydrogen to deuterium in HCOOH (as D 2 O was used as solvent). Reaction time: 148 h. Full size image Table 1 Formic acid formation as function of the catalyst concentration (conc. ), pressure and P (H 2 )/ P (CO 2 ) ratio*. Full size table Under relatively mild conditions (60 °C, 30 bar CO 2 , 30 bar H 2 , 2.76 mM catalyst), [RuCl 2 (PTA) 4 ] hydrogenates CO 2 to afford a 0.03 M formic acid solution. The concentration of formic acid produced depends on the gas pressure. With a P (H 2 )/ P (CO 2 ) ratio of 1 increasing the total gas pressure from 60 bar to 100 bar affords a 0.083 M formic acid solution ( Table 1 ), and at a total gas pressure of 200 bar the concentration of formic acid obtained is 0.204 M ( Fig. 3 ). 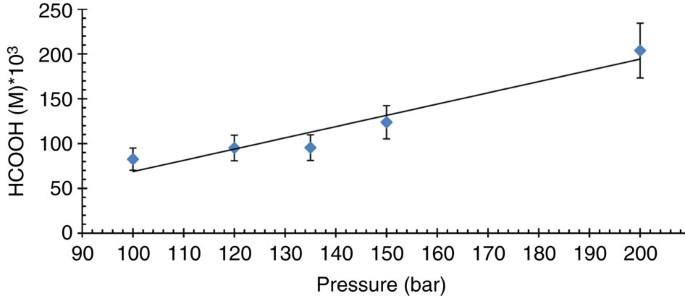Figure 3: Pressure dependence on the concentration of formic acid obtained in the catalytic hydrogenation of CO2. Conditions: the catalyst was dissolved in 2 ml H2O ([RuCl2(PTA)4]=2.76 mM) under N2atmosphere. This solution was pressurized at room temperature with CO2(50 bar) and completed with H2to the desired pressure. The system was heated at 60 °C and stirred until the equilibrium of the reaction was reached (72–96 h). The final yield of formic acid was determined by1H NMR spectroscopy with DSS as an internal standard. The values are averaged from three to six measurements with a reproducibility of ±15%. The trend line is shown as a guide and is not a mathematical fit of the data. Figure 3: Pressure dependence on the concentration of formic acid obtained in the catalytic hydrogenation of CO 2 . Conditions: the catalyst was dissolved in 2 ml H 2 O ([RuCl 2 (PTA) 4 ]=2.76 mM) under N 2 atmosphere. This solution was pressurized at room temperature with CO 2 (50 bar) and completed with H 2 to the desired pressure. The system was heated at 60 °C and stirred until the equilibrium of the reaction was reached (72–96 h). The final yield of formic acid was determined by 1 H NMR spectroscopy with DSS as an internal standard. The values are averaged from three to six measurements with a reproducibility of ±15%. The trend line is shown as a guide and is not a mathematical fit of the data. Full size image The reaction was also studied at temperatures ranging from 23 to 90 °C under standard conditions ([RuCl 2 (PTA) 4 ]=2.76 mM, total pressure=100 bar and P (H 2 )/ P (CO 2 ) pressure ratio=1, see Fig. 4 and Supplementary Fig. 3 and Supplementary Table 2 ). As the hydrogenation of CO 2 is exothermic, increasing temperature reduces the final formic acid concentration, which decreases to 0.032 M at 90 °C. The temperature dependence of the reaction rate follows the Arrhenius law from which activation enthalpy of +96 kJ mol −1 was obtained ( Supplementary Fig. 4 ). 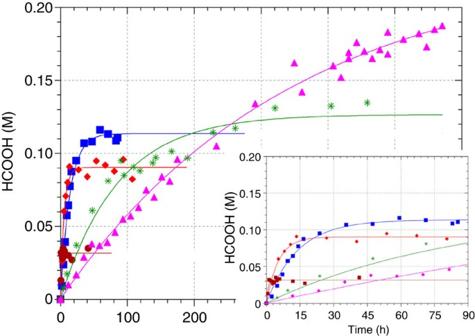Figure 4: Influence of temperature on the hydrogenation of CO2to formic acid using [RuCl2(PTA)4] as the catalyst: 90 °C (brown circle), 60 °C (red diamond), 50 °C (blue square), 40 °C (green asterisk) and 30 °C (pink triangle). Conditions: [RuCl2(PTA)4] was dissolved in H2O (2.76 mM, 2 ml), under N2atmosphere. The solution was pressurized at room temperature with CO2(50 bar) and completed with H2to 100 bar. The system was heated to the desired temperature and the reaction was monitored by1H NMR spectroscopy until the equilibrium of the reaction was reached. The values are averaged from three to six measurements with a reproducibility of ±15%. Figure 4: Influence of temperature on the hydrogenation of CO 2 to formic acid using [RuCl 2 (PTA) 4 ] as the catalyst: 90 °C (brown circle), 60 °C (red diamond), 50 °C (blue square), 40 °C (green asterisk) and 30 °C (pink triangle). Conditions: [RuCl 2 (PTA) 4 ] was dissolved in H 2 O (2.76 mM, 2 ml), under N 2 atmosphere. The solution was pressurized at room temperature with CO 2 (50 bar) and completed with H 2 to 100 bar. The system was heated to the desired temperature and the reaction was monitored by 1 H NMR spectroscopy until the equilibrium of the reaction was reached. The values are averaged from three to six measurements with a reproducibility of ±15%. Full size image Using the optimized catalytic system, recycling experiments were performed and it was found that the catalyst could be reused without the loss of activity ( Supplementary Table 3 ). Carbon dioxide hydrogenation in other solvents As [RuCl 2 (PTA) 4 ] is able to directly hydrogenate carbon dioxide in aqueous acidic solution, that is, at pH=2.70, further studies were performed in water-miscible ionic liquids, that is, 1-butyl-3-methylimidazolium terafluoroborate ([BMIM][BF 4 ]) and 1-butyl-3-methylimidazolium tosylate ([BMIM][tos] where tos=the p -CH 3 C 6 H 4 SO 3 - anion), and in tetrahydrofuran and DMSO ( Table 2 ). Table 2 Catalytic hydrogenation of carbon dioxide to formic acid in different solvent mixtures. Full size table High activities were observed in DMSO/H 2 O with the catalytic activity increasing as the water/solvent ratio was decreased. In pure DMSO at 50 °C, a 1.93 M formic acid solution was obtained at 100 bar with a P (H 2 )/ P (CO 2 ) ratio of 1. Extensive investigations on the activity of [RuCl 2 (PTA) 4 ] in pure organic solvents, that is, alcohols, acetonitrile, propylene carbonate and toluene ( Supplementary Table 4 ), revealed that the catalyst is active in several solvents, although none were as effective as DMSO. 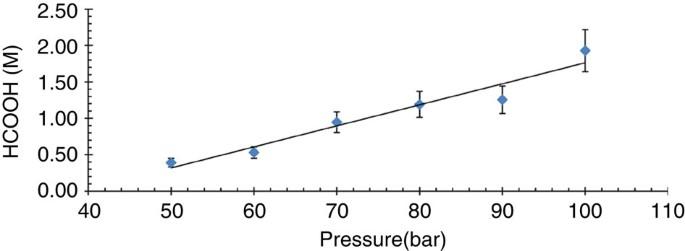Figure 5: Pressure effect on the formic acid yield using [RuCl2(PTA)4] catalyst in DMSO. Reaction conditions: [RuCl2(PTA)4] (2.76 mM),t=50 °C,P(H2)/P(CO2) ratio of 1, reaction time 120 h, DMSO (2 ml), average values of several (two to six) measurements. The trend line is shown as a guide and is not a mathematical fit of the data. Further screening of other catalysts in DMSO ( Supplementary Table 5 ) confirmed the superiority of [RuCl 2 (PTA) 4 ] in the hydrogenation of CO 2 , that is, [RuCl 2 (PTA) 4 ] is ~20 times more active in DMSO compared with the other catalysts evaluated. Hence, the efficiency of [RuCl 2 (PTA) 4 ] in DMSO was studied as a function of the total gas pressure ( Fig. 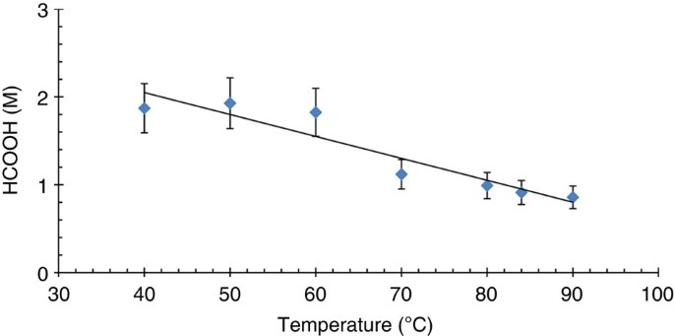Figure 6: The influence of temperature on the hydrogenation of CO2to formic acid using [RuCl2(PTA)4] in DMSO. Conditions: the catalyst was dissolved in 2 ml DMSO ([RuCl2(PTA)4]=2.76 mM) under N2atmosphere. This solution was pressurized at room temperature with CO2(50 bar) and completed with H2to 200 bar (P(H2)/P(CO2)=3). The system was heated to the desired temperature and stirred until the equilibrium of the reaction was reached. The final yield of formic acid was determined by1H NMR spectroscopy with DSS as an internal standard. The trend line is shown as a guide and is not a mathematical fit of the data. The values are averaged from three to six measurements with a reproducibility of ±15%. 5 and Supplementary Table 6 ) and the P(H 2 )/P(CO 2 ) partial pressure. Similar trends were observed to those in water. Figure 5: Pressure effect on the formic acid yield using [RuCl 2 (PTA) 4 ] catalyst in DMSO. Reaction conditions: [RuCl 2 (PTA) 4 ] (2.76 mM), t =50 °C, P (H 2 )/ P (CO 2 ) ratio of 1, reaction time 120 h, DMSO (2 ml), average values of several (two to six) measurements. The trend line is shown as a guide and is not a mathematical fit of the data. Full size image The dependence of the final formic acid concentration and the reaction rate as function of temperature was determined in DMSO ( Fig. 6 , Supplementary Fig. 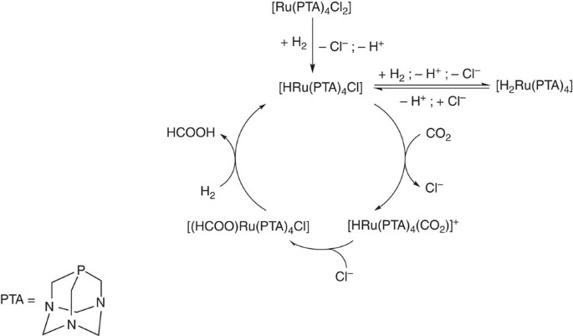Figure 7: Catalytic cycle. Proposed catalytic cycle for the hydrogenation of carbon dioxide using [RuCl2(PTA)4] in water or DMSO. 5 and Supplementary Table 7 ). Similar to the aqueous system, the final formic acid concentration increases as the temperature decreases, whereas the reaction rate increases with increasing temperature. Figure 6: The influence of temperature on the hydrogenation of CO 2 to formic acid using [RuCl 2 (PTA) 4 ] in DMSO. Conditions: the catalyst was dissolved in 2 ml DMSO ([RuCl 2 (PTA) 4 ]=2.76 mM) under N 2 atmosphere. This solution was pressurized at room temperature with CO 2 (50 bar) and completed with H 2 to 200 bar ( P (H 2 )/ P (CO 2 )=3). The system was heated to the desired temperature and stirred until the equilibrium of the reaction was reached. The final yield of formic acid was determined by 1 H NMR spectroscopy with DSS as an internal standard. The trend line is shown as a guide and is not a mathematical fit of the data. The values are averaged from three to six measurements with a reproducibility of ±15%. Full size image The catalyst, [RuCl 2 (PTA) 4 ], was recycled and reused several times ( Table 3 ) without any decrease of activity observed, resulting in a total turn over number (TON) of 749 after four recycles and indicating that considerably higher TONs may be achieved. Table 3 Recyclability of [RuCl 2 (PTA) 4 ] the carbon dioxide hydrogenation in DMSO. Full size table Mechanistic studies with [RuCl 2 (PTA) 4 ] catalyst Moreover, possible catalytic intermediates were identified under catalytic conditions using medium pressure sapphire tubes, by nuclear magnetic resonance (NMR) spectroscopy. The [RuCl 2 (PTA) 4 ] catalyst, both in water and in DMSO-d 6 , together with DSS (4,4-dimethyl-4-silapentane-1-sulphonic acid) as an internal standard, was pressurized to 100 bar with a P (H 2 )/ P (CO 2 ) pressure ratio of 1 and heated at 50 °C. The hydride region of the resulting 1 H NMR spectra reveals the presence of monohydride and dihydride species, that is, [RuH 2 (PTA) 4 ] and [RuH(PTA) 4 Cl], assigned from a multiplet at −11.2 p.p.m. and a doublet of quartets at −9.2 p.p.m., previously observed in aqueous solution ( Supplementary Fig. 6 ) [37] . In the 1 H{ 31 P} NMR spectra, the two hydride signals were shown to collapse into singlet resonances ( Supplementary Fig. 7 ). On the basis of these observations and prior literature [18] , [37] , a tentative catalytic cycle can be proposed ( Fig. 7 ). Figure 7: Catalytic cycle. Proposed catalytic cycle for the hydrogenation of carbon dioxide using [RuCl 2 (PTA) 4 ] in water or DMSO. Full size image The [RuCl 2 (PTA) 4 ] complex catalyses the direct hydrogenation of CO 2 in DMSO to afford formic acid at unprecedentedly high concentrations, that is, 1.9 M (~15% in volume). Importantly, the catalyst operates in the absence of base (or any other additives) and is highly stable and can be recycled and reused without loss of activity. As demand for formic acid continues to grow, notably as a potential hydrogen carrier (HCOOH can selectively decompose into H 2 and CO 2 , Supplementary Figs 8 and 9 ) [38] , [39] , [40] ; viable catalytic processes that directly convert CO 2 into formic acid, such as the one described herein may help to propel a hydrogen-based economy. General considerations NaHCO 3 , NaOH, HCl, HCOOH and sodium 3-(trimethylsilyl)-1-propanesulfonate (DSS) were purchased from Fluka, BASF or Merck. H 2 (99.95%) and CO 2 (99.9%) were acquired from Carbagas-CH, enriched 13 CO 2 (99% in 13 C) was obtained from Cambridge Isotope Laboratories. Double distilled water, DMSO (Sigma-Aldrich), methanol (Fluka), ethanol (Fluka), acetonitrile (Merck), propylene carbonate (Acros), toluene (Merk), ionic liquids [BMIM][BF 4 ] and [BMIM][tos] (Fluka) were used as solvents. Ligands PTA, TPPTS and TPPMS were purchased from ABCR and Fluka, respectively. The ligand MePTA and the complexes [RuCl 2 (PTA) 4 ], [RhCl(TPPMS) 3 ], [RuCl 2 (PTA)([9]aneS 3 )], [Ru(H 2 O) 4 (MePTA) 2 ](tos) 4 , [RuCl 2 (TPPMS) 2 ], [RuCl 2 (TPPTS) 2 ] 2 and [RuCl 2 (p-cymene)] 2 were synthesized according to the literature [41] , [42] , [43] , [44] , [45] , [46] , [47] , [48] , [49] , [50] . All manipulations were carried out under oxygen-free conditions with degassed solvents, using Schlenk line techniques with N 2 as a protective gas. The reactions were carried out in medium pressure sapphire NMR tubes up to 100 bar and were followed by 1 H and 13 C NMR spectroscopy. At higher pressures Parr autoclaves (25 ml, SS 316) were used. NMR spectra were recorded on a Bruker DRX 400 NMR spectrometer and the spectra were fitted with the program WIN-NMR. Formic acid concentrations were determined by quantitative 1 H and 13 C NMR, by ion chromatography using an ICS-90 system and by HPLC with an Agilent 1260 Infinity instrument. Homogeneous catalytic hydrogenation reactions Preliminary studies with different catalysts were performed in a multi-autoclave (HEL CAT 7) by preparing a 2.76 × 10 −3 M (2.76 mM) solution of the corresponding catalyst in degassed water (2 ml). The solutions were then pressurized up to 30 bars of CO 2 and then completed up to 60 bars with H 2 (partial H 2 pressure=30 bar). The system was heated to 60 °C and stirred until the reaction was completed. Formic acid yields were determined by 1 H NMR spectroscopy using DSS as an external standard (c=0.0130 M), and were verified by ionic chromatography and by HPLC. For kinetic measurements, catalysts were dissolved in degassed solvents (2 ml), which were introduced into a sapphire NMR tube or into an autoclave under N 2 atmosphere. The solutions were pressurized up to 20–55 bars with CO 2 and then completed to 60–200 bar with H 2 . The system was heated to the required temperature (23–135 °C) and shaken/stirred. In the sapphire NMR tubes, the evolution of [HCOOH] and [CO 2 ] was followed by quantitative 1 H or 13 C NMR spectroscopy with DSS as an internal standard [51] . For the autoclaves the yield of formic acid was determined by 1 H NMR measurement in the final solution, with DSS as external standard (solution of 0.0130 M), and controlled by ionic chromatography and by HPLC. During the studies using different organic solvents (in which DSS is insoluble), the final formic acid concentrations were determined by 1 H NMR using the standard addition method (with a known [HCOOH] solution), and controlled by ionic chromatography and by HPLC. The dissolved CO 2 and H 2 concentrations were monitored by 13 C and 1 H NMR during the catalytic hydrogenation reactions using medium pressure sapphire NMR tubes [52] , [53] , and display distinct gas and liquid phases under the reaction conditions. Recycling experiments Catalyst recycling experiments were performed using 10 mM [RuCl 2 (PTA) 4 ] solutions in water or in DMSO, with a pressure P (total)=100 bar, P (H 2 )/ P (CO 2 ) ratio of 1, t =60 °C. Once the reaction reached equilibrium, the systems were depressurized, and the formic acid concentrations were determined. The solvent and the formic acid were removed under vacuum and the remaining solid catalyst was dissolved in the appropriate solvent (H 2 O or DMSO), pressurized to 100 bar, P (H 2 )/ P (CO 2 ) ratio of 1. After each reaction, the formic acid concentration was determined by 1 H NMR spectroscopy and the recycling procedure was repeated. In addition, the resulting formic acid could be dehydrogenated into hydrogen and carbon dioxide using an immobilized catalyst described previously [40] . How to cite this article: Moret, S. et al . Direct synthesis of formic acid from carbon dioxide by hydrogenation in acidic media. Nat. Commun. 5:4017 doi: 10.1038/ncomms5017 (2014).